Evidence for the alkaline nature of parental carbonatite melts at Oka complex in Canada The Earth’s sole active carbonatite volcano, Oldoinyo Lengai (Tanzania), is presently erupting unique natrocarbonatite lavas that are characterized by Na- and K-bearing magmatic carbonates of nyerereite [Na 2 Ca(CO 3 ) 2 ] and gregoryite [(Na 2 ,K 2 ,Ca)CO 3 ]. Contrarily, the vast majority of older, plutonic carbonatite occurrences worldwide are dominated by Ca-(calcite) or Mg-(dolomite)-rich magmatic carbonates. Consequently, this leads to the conundrum as to the composition of primary, mantle-derived carbonatite liquids. Here we report a detailed chemical investigation of melt inclusions associated with intrusive (plutonic) calcite-rich carbonatites from the ~120 Ma carbonatite complex of Oka (Canada). Melt inclusions are hosted by magnetite (Fe 3 O 4 ), which crystallizes through a significant period of carbonatite melt solidification. Our results indicate mineral assemblages within the melt inclusions that are consistent with those documented in natrocarbonatite lavas. We propose therefore that derivation of alkali-enriched parental carbonatite melts has been more prevalent than that preserved in the geological record. Carbonatites are igneous rocks consisting of >50% magmatic carbonate minerals, occur on all continents (including Antarctic) and range in age from Archean to present day [1] , [2] . On the basis of experimental data [3] and compilation of their stable (carbon and oxygen) [4] , noble gas (Ne, Xe, Kr, He and Ar) [5] , [6] and radiogenic (Nd, Sr and Pb) isotope data [4] , carbonatite melts are clearly derived from Earth’s upper mantle. The origin of mantle-derived, carbonate-rich liquids remains unresolved, with models varying from direct partial melting of carbonate- and amphibole-bearing mantle [3] , protracted melt differentiation of a carbonated, silica-undersaturated parental melt [7] or via carbonate-silicate liquid immiscibility [8] , [9] . Despite the small number of occurrences worldwide ( n =527) [1] compared with their basaltic counterparts, carbonatites continue to receive considerable deserved attention because of their unique enrichment (relative to crustal abundances) in incompatible trace elements, including the rare earth elements (REEs). These elements are of strategic importance in the continually burgeoning fields of superconductors, electronics and computing. Given their unique geochemical signatures derived from upper mantle sources, widespread tectonic and geographic distribution and emplacement ages that span >3.0 billion years of Earth’s history, these features render carbonatites as insightful probes into deciphering the chemical nature, temporal evolution and metasomatism of Earth’s upper mantle. The >500 carbonatite complexes worldwide are dominated by either Ca- (calcite) or Mg-rich (dolomite) carbonate [1] ; the sole exception being the alkali-rich natrocarbonatite lavas erupted at Oldoinyo Lengai (Tanzania), the only active carbonatite volcano on Earth [10] . This raises the important question as to why most plutonic, older carbonatite complexes worldwide are deficient in alkalis (most notably Na and K), whereas the present-day natrocarbonatite lavas being erupted at Oldoinyo Lengai are enriched in the latter. Hence, there is considerable debate as to the petrogenetic significance of the natrocarbonatites lavas from Oldoinyo Lengai in relation to identifying the chemical composition of parental carbonatite magmas; it is unclear whether these represent the ‘true’ parental carbonatite melts, while the majority of plutonic carbonatite complexes worldwide may have lost their original alkalis by some late-stage or post-magmatic process(es). It is imperative therefore to determine and assess accurately the chemical composition of primitive carbonatite melts, and this may be approached in two ways: first, by examining the nature and chemical composition of melt inclusions within individual minerals present in carbonatites; or second, use of whole rock chemical compositions of carbonatites. However, the latter does not represent parental liquid compositions as they are considered to reflect crystal accumulation [11] , [12] , and may undergo post-crystallization deuteric alteration by late-stage magmatic fluids [13] . In contrast, melt inclusions are: a combination (mechanical mixture) of co-trapped crystals and melt—with the latter typically recrystallizing into daughter crystals; trapped and isolated early in the crystallization history of the magma [14] ; protected by the host mineral from possible low-temperature alteration; and largely excluded from any subsequent reactions or processes within the magma chamber (for example, mixing, degassing, contamination and so on). Hence, melt inclusions represent a powerful tool for determining the chemical composition of parental carbonatite magmas. To date, investigation of melt inclusions associated with intrusive (plutonic) carbonatites are scarce [15] ; however, several investigations have examined melt inclusions in minerals associated with alkali-silicate rocks within carbonatite complexes [16] . Moreover, investigation of melt inclusions for carbonatite complexes located outside of the present-day volcanic activity associated with the East African Rift would prove invaluable as these can serve to test the hypothesis relative to the degree of alkalinity for parental carbonatite melts on a global scale. Here we conduct a detailed, multimineral investigation of melt inclusions associated with intrusive (plutonic) calciocarbonatites from the world renowned 127–115 million year old Oka complex, Canada [17] , located ~40 km west of Montréal, which is one of the most westerly intrusions of the Monteregian Igneous Province [17] . The melt inclusions investigated here are hosted by magnetite, a ubiquitous mineral constituent of carbonatites that typically appears early during both Ca- and Na-rich carbonatite melt differentiation [18] , [19] , [20] . Oka samples and composition of melt inclusions Individual magnetite crystals ( Fig. 1a ; n =449) were embedded in epoxy mounts and, given its opacity during petrographic examination, inclusions were examined on exposed surfaces ( Fig. 1c ). Magnetite from carbonatites at Oka is characterized by relatively high MnO contents (Fe 2 O 3 =63–71 wt%; FeO=16–30 wt%; MnO=4–11 wt%) [21] , and is comparable in composition to those reported for Oldoinyo Lengai (Fe 2 O 3 =62–68 wt%; FeO=11–20 wt%; MnO=11–17 wt%) [20] . The trapped melt inclusions examined in this study are all polycrystalline and contain a complex and varied assemblage of daughter mineral phases (for example, Figs 1c and 2 ). The inclusions are interpreted as trapped melt from which the minerals have crystallized ‘ in situ ’. Their relative proportion is completely random and dependent on the bulk composition of the entrapped melt and on the particular ‘cut’ through the polycrystalline assemblage. Given that the magnetite crystals were taken from 12 individual samples of carbonatite, which encompass the main carbonatite varieties at Oka, we believe that the mineral assemblages recorded within the melt inclusions reported here are representative for the entire complex. Mineral phases have been identified using petrographic microscopy, scanning electron microscopy coupled with energy dispersive X-ray spectroscopy analysis, laser Raman microspectroscopy and electron microprobe (wavelength dispersive spectrometer; WDS) analysis ( Tables 1 and 2 ). 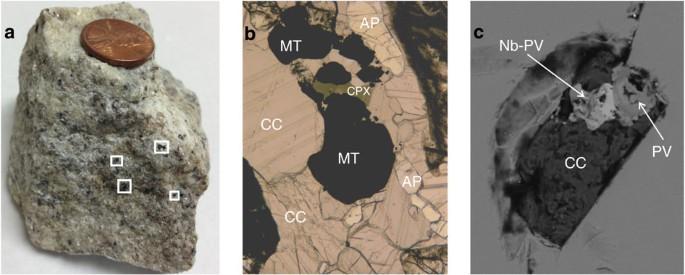Figure 1: Petrographic and mineralogical textural relationships of magnetite within Oka carbonatite. (a) Hand specimen of calciocarbonatite from Oka that contains ubiquitous magnetite crystals (these are highlighted within white boxes); (b) photomicrograph of carbonatite petrographic thin section illustrating the co-crystallization of magnetite with calcite and apatite (field of view is 2.3 cm); (c) a back scatter electron image of a magnetite-hosted, single melt inclusion exposed at the surface (field of view is 200 μm). CC, calcite; MT, magnetite; AP, apatite; PV, pervoskite; Nb-PV, Nb-enriched perovskite; CPX, clinopyroxene. Figure 1: Petrographic and mineralogical textural relationships of magnetite within Oka carbonatite. ( a ) Hand specimen of calciocarbonatite from Oka that contains ubiquitous magnetite crystals (these are highlighted within white boxes); ( b ) photomicrograph of carbonatite petrographic thin section illustrating the co-crystallization of magnetite with calcite and apatite (field of view is 2.3 cm); ( c ) a back scatter electron image of a magnetite-hosted, single melt inclusion exposed at the surface (field of view is 200 μm). CC, calcite; MT, magnetite; AP, apatite; PV, pervoskite; Nb-PV, Nb-enriched perovskite; CPX, clinopyroxene. 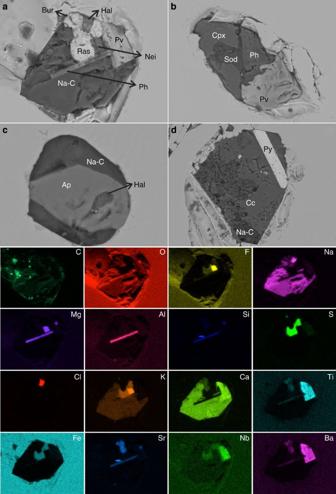Figure 2: Back scatter electron and energy dispersive spectroscopy X-ray images of melt inclusions. (a–d) Represent backscattered electron images of exposed melt inclusions within host magnetite. Energy dispersive X-ray spectroscopy X-ray chemical (elemental) maps (C, O, F, Na, Mg, Al, Si, S, Cl, K, Ca, Ti, Fe, Sr, Nb and Ba) in the lower half of the figure correspond to those for melt inclusion shown ina. AP, apatite; Bur, burbankite; CC, calcite; CPX, clinopyroxene; Hal, halite; Na-C, Na-K-Ca carbonate; Nei, neighborite; Ph, phlogopite; Pv, perovskite; Py, pyrrhotite; Ras, rasvumite; Sod, sodalite. Field of view:a, 60 μm;b, 90 μm;c, 30 μm andd, 125 μm. Full size image Figure 2: Back scatter electron and energy dispersive spectroscopy X-ray images of melt inclusions. ( a – d ) Represent backscattered electron images of exposed melt inclusions within host magnetite. Energy dispersive X-ray spectroscopy X-ray chemical (elemental) maps (C, O, F, Na, Mg, Al, Si, S, Cl, K, Ca, Ti, Fe, Sr, Nb and Ba) in the lower half of the figure correspond to those for melt inclusion shown in a . AP, apatite; Bur, burbankite; CC, calcite; CPX, clinopyroxene; Hal, halite; Na-C, Na-K-Ca carbonate; Nei, neighborite; Ph, phlogopite; Pv, perovskite; Py, pyrrhotite; Ras, rasvumite; Sod, sodalite. Field of view: a , 60 μm; b , 90 μm; c , 30 μm and d , 125 μm. Full size image Table 1 Solid phases in melt inclusions and occurrence distribution. Full size table Table 2 Representative compositions of carbonates in melt inclusions. Full size table The majority of solid phases present in the melt inclusions from Oka ( Table 1 ) are different carbonate minerals (for example, calcite, dolomite, nyerereite and shortite), halides (for example, halite, sylvite and neighborite), sulphates (for example, barite), sulphides (for example, sphalerite) and an admixture of phosphates (apatite), oxides and silicates. Figure 2a provides an example of the various minerals present within a single inclusion, including minerals such as shortite, halite, perovskite, phlogopite, burbankite, neighborite and rasvumite; the presence of these minerals clearly indicates derivation from a melt enriched in the following elements: Na, K, Cl, F, S, Sr and REEs. This assemblage of minerals is similar to that present in the natrocarbonatites of Oldoinyo Lengai, which includes nyerereite, fluorite, apatite-(CaF), barite, magnetite, khanneshite, monticellite and sphalerite. To our knowledge, our study is the first to report the presence of an alkali-rich mineral association and large variety of daughter minerals in melt inclusions from a plutonic, older CaCO 3 -dominated carbonatite complex outside the East African Rift. The relative distribution (% occurrence based on counting statistics) of each type of mineral phase is listed in Table 1 , and these were randomly distributed amongst the different carbonatite samples ( n =12) investigated here. Similar mineral associations have been identified only in two principal rock types: natrocarbonatites [22] , and groundmass, chloride-carbonate and diamond inclusions, and olivine and Cr-spinel hosted inclusions within kimberlites [23] , [24] , [25] , [26] , [27] . Guzmics et al. [12] recently examined the melt inclusions associated with the extrusive (volcanic) calciocarbonatites at Kerimasi volcano (Tanzania), and their results indicate that the carbonatite melt fraction contained between 10 and 20 wt% Na 2 O and K 2 O. Kerimasi is located several kilometres from Oldoinyo Lengai and therefore the alkali-rich nature of its carbonatites is not surprising. Nyerereite is a major mineral within the natrocarbonatite lavas from Oldoinyo Lengai volcano [28] , and has been identified in calciocarbonatite from the Kerimasi volcano [29] . Earlier studies have reported the presence of Na-K-Ca carbonates as inclusions in perovskite and calzirtite from the Guli intrusive Ca-carbonatite, polar Siberia [30] ; perovskite and melilite from Gardiner complex, southeastern Greenland [31] ; melilite from Monte Vulture volcano, Italy [32] ; calcite from the Kerimasi complex, Tanzania [12] ; perovskite from carbonatite lavas, Tinderet volcano (Kenya) [33] ; and fluorite-rich carbonatites from the Bol’shaya Tagna Massif, Russia [15] . The majority of the alkali-enriched carbonates identified in the melt inclusions from Oka define compositions between nyerereite and shortite ( Table 2 ). Compared with carbonate mineral compositions from other carbonatite complexes worldwide, the Na-K-Ca carbonates from Oka contain the highest K contents, with some comparable to those recorded within nyerereite from Oldoinyo Lengai [28] ( Table 2 ). Kogarko et al. [30] suggested that the enrichment of alkalis in the Guli intrusive calciocarbonatite is a derivative from primary calc-alkaline carbonate melts. In contrast, Le Bas [34] argued that natrocarbonatitic magma is the primary melt for Ca- and Mg-rich carbonatites. Dawson [22] supported this latter interpretation by stating that some premodern calciocarbonatite lavas and pyroclastic material containing Na-K-Ca carbonates may have erupted as alkali carbonatite but were subsequently leached of their alkalis. ‘Fenite’ metasomatic aureoles marking expulsion of alkali-rich fluids from carbonatite into the country rocks are common amongst Ca- and Mg-rich carbonatites within intrusive complexes [35] . It is possible, therefore, that formation of calciocarbonatites can be attributed to the loss of alkalis during melt evolution and crystallization, such as during fenitization of the country rocks [34] . Moreover, the source of alkalis within carbonatite liquids must be of mantle origin as Na- and K-metasomatic alteration (fenitization) of the surrounding country rocks is identical in nature regardless of whether these occur in an oceanic setting (for example, Cape Verde and Canary Islands) or continental areas [34] . Veksler et al. [36] proposed a model involving combined crystal fractionation and alkali partitioning into an evolving aqueous fluid phase, which leads to the formation of calcite and associated cumulates that are subsequently surrounded by alkali-rich metasomatic zones (for example, Kovdor and Gardiner carbonatite complexes). The alkali-rich carbonate component could be easily replaced by secondary calcite at atmospheric conditions within a matter of days [37] . The loss of alkalis and other elements (for example, REE, Cl) from silicate-hosted calcite and dolomite globules has also been documented in tuffs during syn- and post-magmatic alteration [38] . The results and conclusions presented here are supported by the experimental data from Kjarsgaard [39] , which suggest that a minimum of ~5–7 wt% of (Na 2 O+K 2 O) is present in carbonatite melts produced at pressures between 0.2 and 0.5 GPa (these correspond to crustal levels). In addition, the experimentally quenched sodic dolomitic carbonatite liquids produced at high temperature (930–1,030 °C) and high pressure (21–30 kbar) by Wallace and Green [3] contain 0.5% P 2 O 5 , 3% SiO 2 , 2% Al 2 O 3 , 5% FeO, 5% Na 2 O and 0.4% K 2 O, which allow for the crystallization of the non-carbonate minerals (for example, phosphates, oxides and silicates). These experimental results indicate that alkalis may be involved in the generation of carbonate melts at upper mantle conditions, and that the latter are enriched in alkalis relative to Na and K abundances reported in the majority of Ca-rich carbonatites worldwide. Moreover, Gittins [7] pointed out that silicon, aluminium, phosphorus and iron (in addition to Na and K) are necessary to produce the variety of trace phosphate, silicate and oxide minerals coexisting with calcite and dolomite in carbonatites. Le Bas [34] indicated that the sources of Na and K in primary carbonatite liquids may be acquired during partial melting of an amphibole- or phlogopite-bearing mantle, respectively; with the ultimate Na:K ratio of the carbonatite melt dependent on the mineralogy of the mantle source. On the basis of the mineral assemblages and compositions within melt inclusions reported here, it is difficult to reconstruct the exact (bulk) composition of the ‘primitive’ alkali-rich carbonatite liquid as the crystallization history of magnetite is extensive, and it may not necessarily be a liquidus phase [18] . Thus, there is a possibility that the trapped liquids (and corresponding daughter crystals) may represent derivative compositions; however, this does not detract from the main finding of our study in that the precursor carbonatite liquid at Oka was alkali rich. It is also challenging to determine exact volumes and reconstruct bulk liquid compositions based on mineral compositions, as inclusions may be present both above and below the exposed surface in the magnetite crystals. The melt inclusions investigated here represent random sections of heterogeneously trapped crystals and recrystallized melt; this renders homogenization (that is, quenching) experiments of the inclusions by heating somewhat futile. On the basis of the melt inclusion results reported in this study, we argue that the parental carbonatite liquid at Oka was alkali rich, and thus provides some direct evidence for the more pervasive occurrence of Na- and K-rich carbonatite liquids on a global scale. The data presented here suggest that natrocarbonatite-like parental melts are not simply restricted to the modern occurrences of carbonatites confined to the East African Rift (for example, Oldoinyo Lengai and Kerimasi) but rather occurred in the geological past and in different continental rift areas. Sample preparation Magnetite grains were magnetically separated from crushed rock samples, optically selected and mounted in epoxy resin. The mounts are prepared using kerosene as a lubricant to prevent loss of water-soluble components or hydration of phases present. Subsequent to exposure, the samples were platinum coated and stored in a desiccator to avoid interaction with atmospheric moisture. Phase identification Backscattered electron imaging and elemental mapping were conducted with a Hitachi SU-70 Schottky field emission scanning electron microscope fitted with Oxford INCA Energy XMax 80 silicon drift detector energy dispersive X-ray spectroscopy system operated at 7 kV and 1 nA at the University of Tasmania (Australia). Carbonates and sulphates were further confirmed using a Renishaw inVia Raman microscope with streamline plus and coupled with a Rencam charge-coupled device camera at the University of Tasmania. Wavelength (633 nm) and a laser power of 10 or 50 mJ per pulse at grating of 1,200 cm −1 were used for sample excitation. All spectra were measured in the high-frequency range between 100 and 1,340 cm −1 . Composition determination Electron microprobe analysis-WDS of solid phases for carbonatite melt inclusions was performed with a Cameca SX100 electron microprobe equipped with a tungsten filament and five spectrometers at the University of Tasmania. The analytical conditions were as follows: accelerating voltage at 15 kV, beam current at 10 nA and focused beam diameter of 3–10 μm depending on mineral size. Na volatilization of carbonates during electron microprobe analysis was monitored and corrected for using a time-dependent correction algorithm (based on time versus counts per second behaviour); this correction was also applied for the measured intensities of K, F, Cl and Fe. CO 2 contents for carbonates were calculated based on cation stoichiometry and included in the matrix correction. The in-house Railton Calcite standard was used for calibration purposes. Interference and matrix (ZAF: atomic number-absorption-fluorescence method) corrections are from Donovan et al. [40] and Armstrong [41] , respectively. How to cite this article: Chen, W. et al. Evidence for the alkalic nature of parental carbonatite melts at Oka complex in Canada. Nat. Commun. 4:2687 doi: 10.1038/ncomms3687 (2013).